Gene co-expression network analysis reveals common system-level properties of prognostic genes across cancer types Prognostic genes are key molecules informative for cancer prognosis and treatment. Previous studies have focused on the properties of individual prognostic genes, but have lacked a global view of their system-level properties. Here we examined their properties in gene co-expression networks for four cancer types using data from ‘The Cancer Genome Atlas’. We found that prognostic mRNA genes tend not to be hub genes (genes with an extremely high connectivity), and this pattern is unique to the corresponding cancer-type-specific network. In contrast, the prognostic genes are enriched in modules (a group of highly interconnected genes), especially in module genes conserved across different cancer co-expression networks. The target genes of prognostic miRNA genes show similar patterns. We identified the modules enriched in various prognostic genes, some of which show cross-tumour conservation. Given the cancer types surveyed, our study presents a view of emergent properties of prognostic genes. Prognostic genes have properties (such as expression level or mutation status) that are informative regarding clinical outcomes. These genes are of particular biomedical interest in cancer research because of their potential as biomarkers, to help predict patients’ survival, and to provide insights into the molecular mechanisms of tumour progression [1] , [2] , [3] , [4] , [5] . Over the past decades, tremendous efforts have been made to identify prognostic genes and build more effective models for stratifying individuals with cancer [6] , [7] , [8] , [9] , [10] , [11] . However, such studies have focused on individual prognostic genes and their clinical utilities, without investigating the emergent properties and behaviours of prognostic genes at the system level. Biological networks represent valuable platforms for understanding system-level properties [12] , [13] , [14] . The commonly used biological networks include protein–protein interaction networks, signalling networks, metabolic networks, gene regulatory networks and gene co-expression networks. Compared with other types of biological networks, using gene co-expression networks has several advantages [15] : nearly complete coverage of human genes, little bias due to the knowledge obtained from the published literature, and the ability to construct cancer-type-specific networks. Using recently available cancer genomic data from ‘The Cancer Genome Atlas’ (TCGA), we investigated the properties of prognostic genes in the gene co-expression networks of four representative cancer types (glioblastoma multiforme (GBM), ovarian serous cystadenocarcinoma (OV), breast invasive carcinoma (BRCA) and kidney renal clear cell carcinoma (KIRC)) [16] , [17] , [18] , [19] . Here we focused on three primary questions about expression-based prognostic genes. First, are there network properties that distinguish prognostic genes from other genes in the co-expression networks? Second, do different types of prognostic genes show similar network properties? Third, do those patterns hold true across different cancer types? We performed a comparative analysis of prognostic genes in terms of key network properties (for example, whether they tend to be hub genes and enriched in modules) across the four cancer types. Our results reveal some common and distinct patterns of prognostic genes and identify modules associated with prognostic signatures. This study contributes to a comprehensive understanding of the informative behaviours of prognostic genes from the point of view of systems biology. Prognostic mRNA genes tend not to be hub genes In this study, we focused on the four TCGA cancer types with adequate follow-up/survival data and sufficient sample size. The power of detecting prognostic genes varies from one cancer to another, which mainly depends on the sample size and the number of survival events (that is, death). Here we defined prognostic genes as those whose mRNA expression levels are significantly correlated with overall patient survival in two alternative ways: first, different numbers of prognostic mRNAs were identified based on the signal-to-noise ratio within each sample cohort; and second, the top 1,000 mRNA genes most correlated with patient survival were identified per cancer type. We obtained very similar results using these two strategies, and throughout the text, we will mainly present the results based on the first method. With the first method, we identified 1,706, 728, 974 and 2,050 prognostic mRNA genes in GBM, OV, BRCA and KIRC, respectively ( Fig. 1a , Methods). These prognostic genes showed great robustness through the assessment of subset samplings (Methods, Supplementary Fig. 1a ), and the four cancer types shared only a small portion (3–12%) of these prognostic genes ( Supplementary Fig. 1b ). For each cancer type, we constructed a gene co-expression network from Agilent microarray data using weighted gene correlation network analysis (WGCNA) [20] , [21] . WGCNA is a well-established method designed for constructing co-expression networks from microarray-based expression data, and considers not only the co-expression patterns between two genes but also the overlap of neighbouring genes. As a result, we obtained four cancer-type-specific co-expression networks, each containing the same set of 17,813 genes (nodes). These co-expression networks are weighted networks in which any two nodes are connected with an edge weight (from 0 to 1, where 0 indicates no interaction and 1 a strong interaction). Previous studies have indicated that a weighted network retains more information and is more robust and accurate than an unweighted one in network analysis [15] , [21] . 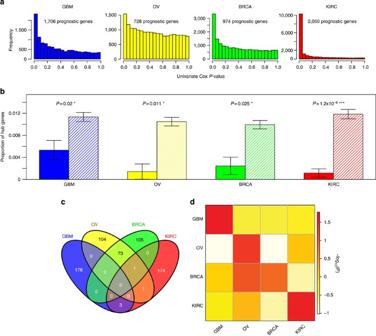Figure 1: The depletion of prognostic mRNA genes in hubs. (a) TheP-value distributions of the correlations of mRNA expression with overall survival based on the univariate Cox model in the four cancer types. Based on the signal-to-noise ratio, prognostic mRNA genes were identified. (b) Prognostic mRNA genes are depleted in the hubs. Solid bars represent the proportions of hub genes among prognostic mRNA genes; striped bars represent the proportions of hub genes among non-prognostic mRNA genes. Error bars indicate±1 s.e.m., andP-values were calculated based on Fisher’s exact tests. (c) The Venn diagram of hub genes across the four cancer types. (d) The heatmap showing the cancer-type-specific pattern of hub depletion. The colour of each cell represents the depletion score of prognostic mRNA genes of a cancer type (column) in hub genes of another cancer type (row); row-wise scaled −log10(P-value) is plotted with red indicating significant, white indicating not significant.P-values were calculated based on Fisher’s exact tests. Figure 1: The depletion of prognostic mRNA genes in hubs. ( a ) The P -value distributions of the correlations of mRNA expression with overall survival based on the univariate Cox model in the four cancer types. Based on the signal-to-noise ratio, prognostic mRNA genes were identified. ( b ) Prognostic mRNA genes are depleted in the hubs. Solid bars represent the proportions of hub genes among prognostic mRNA genes; striped bars represent the proportions of hub genes among non-prognostic mRNA genes. Error bars indicate±1 s.e.m., and P -values were calculated based on Fisher’s exact tests. ( c ) The Venn diagram of hub genes across the four cancer types. ( d ) The heatmap showing the cancer-type-specific pattern of hub depletion. The colour of each cell represents the depletion score of prognostic mRNA genes of a cancer type (column) in hub genes of another cancer type (row); row-wise scaled −log 10 ( P -value) is plotted with red indicating significant, white indicating not significant. P -values were calculated based on Fisher’s exact tests. Full size image One key property for a gene in a biological network is connectivity, which reflects how frequently a node interacts with other nodes (for a weighted network, connectivity is defined as the sum of the weights across all edges of a node). According to the node connectivity, genes can be further classified into hub genes (with an extremely high level of connectivity) and non-hub genes. Hub genes are very important nodes, and in the protein interaction networks of various organisms, hub proteins tend to encode essential genes [22] , [23] , [24] . In the gene co-expression network, hub genes represent a small proportion of nodes with maximal information exchange with other nodes. For example, one prognostic hub gene in GBM is KLKL1 , which is a serine protease with diverse physiological functions. We first examined the properties of connectivity and enrichment for the prognostic genes. We found that, on average, prognostic genes have higher connectivity, but this association does not follow a simple monotonic increasing trend. The prognostic genes appeared to be depleted in nodes with either extremely low or high connectivity ( Supplementary Fig. 2 ). To formally test whether prognostic genes are less likely to be hub nodes in the co-expression networks, we examined the connectivity distributions and defined the 1% (or 5%) of nodes with the highest connectivity as hub genes, according to the literature [25] , [26] , [27] . We found that prognostic genes are significantly depleted in the hubs across all four cancer types ( Fig. 1b ; Supplementary Fig. 3 includes the bar plots of a random same-size set of non-prognostic genes for comparison; Supplementary Fig. 4 ). In addition, we observed the same patterns when the top 1,000 prognostic gene sets were used ( Supplementary Fig. 5 ). In general, the hub genes defined in the different cancer networks are highly specific and show only a little overlap, except that OV and BRAC share some hub genes due to their pathophysiological similarity ( Fig. 1c ). To further examine whether the observed depletion of prognostic genes in hubs is unique to the cancer-specific network, we performed similar analyses using prognostic genes and hub genes defined in different co-expression networks. Figure 1d shows the results in a heatmap format: significant depletions were primarily observed along the diagonal line, demonstrating that prognostic genes in one cancer type show a significant depletion in only the hubs of the corresponding co-expression network. Prognostic mRNA genes are enriched in modules Another important aspect of a gene co-expression network is modularity: genes that are highly interconnected within the network are usually involved in the same biological modules or pathways [28] , [29] . Using WGCNA, we defined the modules in each cancer co-expression network ( Fig. 2a , Methods), and detected 85, 98, 55 and 81 modules in GBM, OV, BRCA and KIRC, respectively. For example, one common module across tumour types is enriched with genes related to the regulation of cell death and apoptosis. The corresponding proportions of module genes are 36.9, 34.7, 26.5 and 29.6% in these cancer types. Strikingly, except for BRCA, prognostic mRNA genes show a significant enrichment in modules ( Fig. 2b ; Supplementary Fig. 6 includes the bar plots of a random same-size of non-prognostic genes for comparison). Moreover, we obtained the same patterns using the top 1,000 prognostic gene sets ( Supplementary Fig. 5d ). In contrast to hub genes, there is substantial overlap of module genes across tumour types ( Fig. 2c ). This is reasonable since modules largely reflect the underlying biological processes. 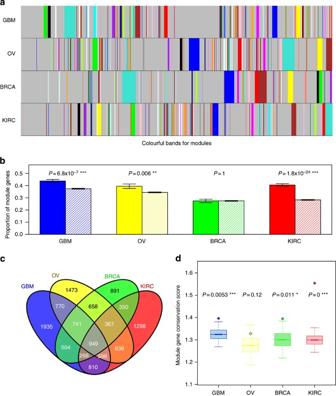Figure 2: The enrichment of prognostic mRNA genes in modules. (a) Modules defined from the weighted gene co-expression networks. Colourful bands represent modules in the network, with the biggest module in turquoise, second largest in blue, then brown, green, yellow and so on. (b) Prognostic genes are enriched in the modules. Solid bars represent the proportions of module genes among prognostic mRNA genes; striped bars represent the proportions of module genes among non-prognostic mRNA genes. Error bars indicate±1 s.e.m., andP-values were calculated based on Fisher’s exact tests. (c) The Venn diagram of module genes across the four cancer types. (d) Boxplots (median±1 quartile, with whiskers extending to the most extreme data point within one interquartile range from the box boundaries) showing that prognostic genes tend to be more conserved module genes.yaxis represents the module-gene conservation score, which ranges from 0 to 4, with 0 indicating not a module gene in any of the four cancer types and 4 indicating a module gene in all four cancer types. Each boxplot represents the mean-conservation-score distribution of 20,000 randomly sampled same-size gene sets; the diamond dot represents the mean conservation score of prognostic genes.P-values were calculated based on Wilcoxon rank sum tests. Figure 2: The enrichment of prognostic mRNA genes in modules. ( a ) Modules defined from the weighted gene co-expression networks. Colourful bands represent modules in the network, with the biggest module in turquoise, second largest in blue, then brown, green, yellow and so on. ( b ) Prognostic genes are enriched in the modules. Solid bars represent the proportions of module genes among prognostic mRNA genes; striped bars represent the proportions of module genes among non-prognostic mRNA genes. Error bars indicate±1 s.e.m., and P -values were calculated based on Fisher’s exact tests. ( c ) The Venn diagram of module genes across the four cancer types. ( d ) Boxplots (median±1 quartile, with whiskers extending to the most extreme data point within one interquartile range from the box boundaries) showing that prognostic genes tend to be more conserved module genes. y axis represents the module-gene conservation score, which ranges from 0 to 4, with 0 indicating not a module gene in any of the four cancer types and 4 indicating a module gene in all four cancer types. Each boxplot represents the mean-conservation-score distribution of 20,000 randomly sampled same-size gene sets; the diamond dot represents the mean conservation score of prognostic genes. P -values were calculated based on Wilcoxon rank sum tests. Full size image To further examine the relationships between prognostic genes and modules in the co-expression networks, for each gene, we calculated a module-gene conservation score (range 0–4), which indicates how frequently a gene is classified in a module among the four cancer types. We found that the conservation scores of prognostic genes are significantly higher than those of other genes in GBM, BRCA and KIRC; the same trend holds true in OV, but with a marginal significance ( Fig. 2d ). These results indicate that prognostic mRNA genes are enriched in module genes, especially in conserved module genes. Target genes of prognostic microRNAs show similar patterns In addition to prognostic mRNA genes, we examined the network properties of prognostic miRNA genes, an important class of non-coding regulatory genes [30] , [31] . Similar to prognostic mRNAs, we defined prognostic miRNA genes based on the correlations of their expression levels with overall patient survival in two ways: first, different numbers of prognostic miRNAs were identified based on the signal-to-noise ratio within each sample cohort; and second, the top 50 miRNA genes most correlated with patient survival were identified per cancer type. We obtained very similar results using these two methods, and will mainly focus on the results from the first method. We identified 15, 106, 54 and 203 prognostic miRNAs in GBM, OV, BRCA and KIRC, respectively ( Fig. 3a , Methods). Since the gene co-expression networks consist of mRNA genes only, we investigated the properties of the target genes of the prognostic miRNAs identified by a leading miRNA target prediction programme, TargetScan [32] . Strikingly, we observed the same patterns: the target genes of prognostic miRNAs are depleted in hub genes ( Fig. 3b ; Supplementary Fig. 7 shows the results when the 5% of nodes with the highest connectivity were defined as hub genes). Considering the noise in miRNA target prediction, we further examined the predicted targets of prognostic miRNAs with different stringent criteria and obtained concordant results ( Supplementary Fig. 8 , Methods). We also obtained the same results using the top 50 prognostic miRNA sets ( Supplementary Fig. 9 ). Moreover, the target genes of prognostic miRNAs are more likely to be enriched in modules than those of non-prognostic miRNAs ( Fig. 3c ; Supplementary Fig. 9d shows the results for the top 50 prognostic miRNA sets). These results suggest that prognostic mRNA and miRNA genes share similar network properties in the cancer gene co-expression networks. 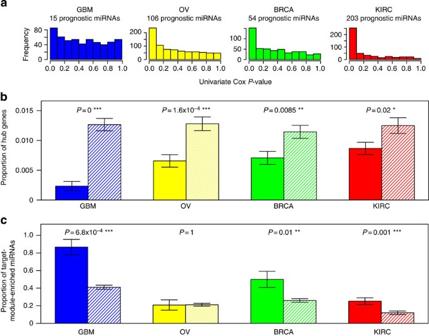Figure 3: Target genes of prognostic miRNA genes show the same patterns. (a) TheP-value distributions of the correlations of miRNA expression with overall survival based on the univariate Cox model in the four cancer types. Based on the signal-to-noise ratio, prognostic miRNA genes were identified. (b) Target genes of prognostic miRNA genes are depleted in the hubs. Solid bars represent the proportions of hub genes among target genes of prognostic miRNAs; striped bars represent the proportions of hub genes among non-target genes of prognostic miRNAs. (c) Target genes of prognostic miRNAs are enriched in the modules. Solid bars represent the proportions of target-module-enriched miRNAs among prognostic miRNAs; striped bars represent the proportions of target-module-enriched miRNAs among non-prognostic miRNAs. Error bars indicate±1 s.e.m., andP-values were calculated based on Fisher’s exact tests. Figure 3: Target genes of prognostic miRNA genes show the same patterns. ( a ) The P -value distributions of the correlations of miRNA expression with overall survival based on the univariate Cox model in the four cancer types. Based on the signal-to-noise ratio, prognostic miRNA genes were identified. ( b ) Target genes of prognostic miRNA genes are depleted in the hubs. Solid bars represent the proportions of hub genes among target genes of prognostic miRNAs; striped bars represent the proportions of hub genes among non-target genes of prognostic miRNAs. ( c ) Target genes of prognostic miRNAs are enriched in the modules. Solid bars represent the proportions of target-module-enriched miRNAs among prognostic miRNAs; striped bars represent the proportions of target-module-enriched miRNAs among non-prognostic miRNAs. Error bars indicate±1 s.e.m., and P -values were calculated based on Fisher’s exact tests. Full size image Some prognostic modules are conserved across tumour types Since both prognostic mRNA genes and the targets of prognostic miRNAs are enriched in the modules of co-expression networks, we were also interested in identifying individual prognostic modules and determining their relationships across cancer types. For this purpose, we first identified modules enriched with prognostic mRNA genes (false discovery rate (FDR) <0.1), and found 47 prognostic modules across the four cancers (GBM: 13, OV: 8, BRCA: 8 and KIRC: 18), with module sizes (number of genes within a module) ranging from 21 to 793 ( Fig. 4a , Supplementary Data 1 ). For each cancer type, tumour subtypes classified by the gene expression of these prognostic modules showed distinct survival curves, highlighting their potential clinical relevance (Methods, Supplementary Fig. 10 ). We further annotated their biological themes through gene ontology (GO) terms [33] . The common themes across the four cancers included ‘response to wounding and inflammation,’ ‘regulation of cell death/apoptosis,’ ‘RNA biosynthetic processing,’ ‘translational elongation and termination,’ ‘signalling pathway regulation,’ ‘regulation of kinase cascade,’ ‘cellular response to hormone/chemical stimulus’ and ‘multiple lipids metabolic and biosynthesis process.’ Besides the common themes, there were specific module themes for each cancer type, such as ‘nervous system development,’ ‘negative regulation of gliogenesis,’ ‘type I interferon-mediated signalling pathway’ and ‘response to metal ion’ in GBM; ‘negative regulation of histone modification’ and ‘tRNA aminoacylation for protein translation’ in OV; ‘chromatin remodelling’ and ‘smooth muscle tissue development’ in BRCA, and ‘positive regulate CREB transcription factor activity,’ ‘interleukin-1-mediated signalling pathway,’ ‘negative regulation of WNT receptor signalling pathway’ and ‘stress-activated MAPK cascade’ in KIRC. 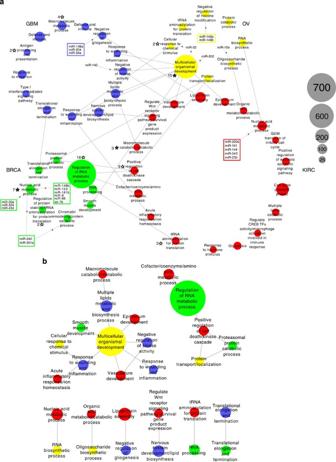Figure 4: Integrative analysis of prognostic modules. (a) The 47 prognostic modules are plotted in four circles, each representing one cancer type. Grey solid lines represent the conservation correspondence between two modules from two different cancer types. Dashed grey lines with black arrow represent the connections of miRNAs whose target genes are enriched in the module. Two or more miRNAs targeting the same module(s) are enclosed within a rectangle; miRNAs as module regulators in more than one cancer type are shown in boldface. Solid black stars mark the modules enriched with significantly mutated pan-cancer genes, and the associated number indicates the number of mutated genes; unfilled black stars mark enrichment that is significant only before multiple testing correction. (b) Plot showing a zoomed-in view of the 22 with cross-tumour modules conservation correspondence in (A). Figure 4: Integrative analysis of prognostic modules. ( a ) The 47 prognostic modules are plotted in four circles, each representing one cancer type. Grey solid lines represent the conservation correspondence between two modules from two different cancer types. Dashed grey lines with black arrow represent the connections of miRNAs whose target genes are enriched in the module. Two or more miRNAs targeting the same module(s) are enclosed within a rectangle; miRNAs as module regulators in more than one cancer type are shown in boldface. Solid black stars mark the modules enriched with significantly mutated pan-cancer genes, and the associated number indicates the number of mutated genes; unfilled black stars mark enrichment that is significant only before multiple testing correction. ( b ) Plot showing a zoomed-in view of the 22 with cross-tumour modules conservation correspondence in (A). Full size image Interestingly, among the 47 prognostic modules, 9 prognostic modules were also enriched with the targets of 23 prognostic miRNAs (FDR<0.1, Fig. 4a ). Among them, three miRNAs ( miR-32 , miR-301a and miR-340 ) show target enrichment in at least two modules, and two miRNAs ( miR-148a and miR-148b ) are associated with prognostic modules in two cancer types. In addition, three prognostic modules are enriched with significantly mutated genes identified in the TCGA Pan-Cancer project (FDR<0.1, Fig. 4a ). To investigate the prognostic modules conserved across tumour types, we determined the module correspondence by considering the members that overlap between the two prognostic modules. This analysis revealed 22 pairwise correspondences among the 47 prognostic modules across the 4 cancers ( Fig. 4b ). Remarkably, one OV module annotated with ‘multicellular organismal development’ acted like a module ‘hub,’ directly linking seven other modules of different cancer types with a wide range of biological themes. In this study, we performed a systematic analysis of the properties of prognostic genes in the context of biological networks across multiple cancer types. Importantly, we used the gene co-expression networks constructed from a single type of microarray as the investigation platform. This practice reduces various confounding factors in the data analysis, such as prior knowledge bias, which occurs from using other types of biological networks or batch effects when constructing the networks from expression data from multiple profiling techniques. Strikingly, although both prognostic genes and hub/module membership in the networks varied greatly from one cancer type to another, our study revealed some distinct properties of prognostic genes. The consistent nature of the patterns we found across multiple cancer types and both prognostic mRNA and miRNA genes (through their target genes) highlights the robustness of the observed pattern. This study provides the first system-level understanding of the ‘informer’ behaviours of cancer prognostic genes, thereby laying a foundation for how to incorporate the co-expression network information into prognostic modelling. For example, since both prognostic mRNAs and miRNAs appear to be preferably associated with some biological modules, on a practical level, further efforts are warranted for building module-based prognostic models, and the models thereby obtained will be more biologically interpretable. Furthermore, the analysis on prognostic modules across tumour types provides a unique perspective to elucidate the common/distinct biological processes involved in different cancer types, which may facilitate novel subtype classifications. Hubs are topologically central in the co-expression network, having maximal informational connections with other genes. Despite prognostic genes having higher connectivity overall, we found them to be depleted in the hub nodes of the cancer-specific co-expression networks. One possible explanation for this finding is that the hubs act more like modulators, coordinating gene expression over many functional components (pathways). As hubs are associated with a very high level of activity of receiving and sending signals, their expression levels are often complicated by too many factors to correlate with the phenotype directly. This observation is compatible with the results from a genomic analysis of the hierarchical structure of gene regulatory networks [34] . Another explanation is that hubs may have more backup and feedback mechanisms to ensure their robust behaviour, so their status may not sensitively reflect the properties of the whole system. In contrast, prognostic genes are enriched in modules, especially in module genes that are conserved across tumour types. Modules in the co-expression network represent groups of functionally related genes dedicated to specific biological processes, which perform essential functions from baseline housekeeping to activities related to tumour growth and invasion. Compared with genes that mainly work alone, the status of a module gene more frequently reflects the ‘group’ behaviour, and is therefore more informative regarding tumour progression. MicroRNAs are an important class of regulatory genes that largely lead to gene silencing through either mRNA degradation or translational inhibition [30] , [31] . Recently, miRNAs have been widely implicated in tumour biology [35] , [36] . The target genes of prognostic miRNAs show patterns similar to those of prognostic mRNA genes in terms of hub and module properties. In particular, we found that some prognostic miRNAs have their target genes enriched in prognostic modules. It is likely that these miRNAs act as a master regulator, coordinating the behaviour of the whole module through their targeting. For example, in GBM, such modules involve functions related to ‘negative regulation of gliogenesis’, ‘negative regulation of kinase activity’ and ‘nervous system development and functions’, all of which are connected with the normal function and development of the brain. Compared with single prognostic genes, biological modules enriched with prognostic genes may represent more robust prognostic signatures, and deserve further investigation. Our integrative analysis reveals several such modules of particular interest. In GBM, the module of ‘negative regulation of gliogenesis’ ( Fig. 4a ) shows an enrichment of target genes of three prognostic miRNAs ( miR-148a , miR-204 and miR-34a ). In terms of the Ingenuity Pathway Analysis (IPA) disease annotation, ‘tumorigenesis of neuroendocrine carcinoma’, ‘recurrence of carcinoma’ and ‘squamous-cell carcinoma’ are the top three terms. Interestingly, the upstream transcription regulators of this module ( ZNF217 , ASCL1 , DNAJB6 , DEK and E2F5 ) are also the predicted targets of the three prognostic miRNAs. In BRCA, there are two prognostic modules regulated by prognostic miRNAs. One is annotated as ‘nucleic acid metabolic process’ ( Fig. 4a ). This module is enriched with the target genes of several prognostic miRNAs ( miR-30a , miR-324 , miR-454 , miR-340 , miR-301a , miR-148b , miR-153 , miR-181b , miR-9 , miR-98 and let-7b ) associated with IPA terms ‘cell death and survival, cell cycle, cancer’ and the oestrogen receptor signalling pathway. It also shows an enrichment of significantly mutated pan-cancer genes ( KIAA1109 , NCOA3 , TAF1 , EP300 , SETD2 , STAG2 and TAF1L ). Thus, this module appears to integrate multiple types of aberration signatures and likely plays an important role in the progression of breast cancer. Another BRCA module associated with prognostic miRNAs is annotated as ‘chromatin remodelling’ and ‘protein catabolic process’ ( Fig. 4a ), suggesting a key role of epigenetic modification in breast cancer. This module is associated with the AMPK signalling pathway, a known oncogenic signalling pathway in breast cancer [37] , [38] . In KIRC, one module annotated as ‘nucleic acid metabolic process’ ( Fig. 4a ) has connections with five prognostic miRNAs. In OV, the module of particular interest is annotated as ‘multicellular organismal development.’ The top IPA disease terms include ‘endometrial cancer’, ‘uterine serous papillary cancer’, ‘epithelia neoplasia’, ’metastatic colorectal cancer’ and ‘solid tumour’, and the enrichment of ‘ovarian adenocarcinoma’ is also significant ( P <1 × 10 −5 , Fisher's exact test). This module is also enriched with significantly mutated pan-cancer genes ( APC , NAV3 , COL11A1 , TSHZ3 , CDH1 , RUNX1 , AR , SYNE1 , MN1 , DCHS1 , PDGFRA , TGFBR2 , CDKN1A , ABCA9 and TNFAIP6 ). Interestingly, this module shows correspondence to quite a few prognostic modules in other cancer types ( Fig. 4b ). Thus, we speculate that this module may reflect a theme that is common across many cancer types. Further investigation is required to evaluate the clinical utility of these modules, such as in patient prognosis stratification and tumour subtype classification. While our study provides some insight into the emergent properties of prognostic genes, more efforts are required to validate and extend our findings. We examined the properties of prognostic genes in the context of gene co-expression networks. A logical extension of this work would be to determine whether the observed patterns hold true in other biological networks, such as protein interaction networks or gene regulatory networks. A major challenge for that direction is that those networks are usually highly biased toward well-studied genes. A second logical extension would be to determine whether the same patterns hold true in the co-expression networks of other tumour types or diseases. Our findings are based on TCGA data, so a third and critical extension of this work would be to learn whether the patterns can be recapitulated by other independent sample cohorts with adequate survival data. Finally, future efforts should be made to incorporate this system-level understanding of prognostic genes into the practice of building effective prognostic models. Identification of prognostic mRNA and miRNA genes We obtained TCGA gene expression and overall survival data from Firehose ( https://confluence.broadinstitute.org/display/GDAC/Home ) and TCGA Pan-Cancer website ( http://pancancer.soe.ucsc.edu/ ). All data are from pan-cancer 4.0 Freeze version. We detected prognostic mRNA or miRNA genes based on the raw Wald P -values generated from the univariate Cox model. We used two methods to define prognostic genes. First, depending on the signal-to-noise ratio, different FDRs were applied: for mRNA genes, 1,706 genes in GBM ( P <0.028, FDR<0.2), 728 genes in OV ( P <0.019, FDR<0.5), 974 genes in BRCA ( P <0.0053, FDR<0.1) and 2,050 genes in KIRC ( P <2.24 × 10 −6 , FDR<2 × 10 −5 ); for miRNA genes, 15 miRNAs in GBM ( P <0.0053, FDR<0.2), 106 miRNAs in OV ( P <0.026, FDR<0.2), 54 miRNAs in BRCA ( P< 0.01, FDR<0.1) and 203 miRNAs in KIRC ( P <0.043, FDR<0.1). We assessed the robustness of these prognostic genes through randomly sampled subsets: based on 100 subsets (75% of the original sample size), on average, 75.3, 75.0, 92.0 and 99.9% of the prognostic mRNA genes showed significant survival correlations in GBM, OV, BRCA and KIRC, respectively ( Supplementary Fig. 1 ). Second, the top 1,000 mRNAs or top 50 miRNAs most correlated with overall survival were identified as prognostic genes. When gene or miRNA expression data were available from more than one platform (Agilent 244 K microarray and Illumina HiSeq RNA-seq), we compared the Wald P -value distributions between the platforms and chose the one with a better signal-to-noise ratio ( Table 1 and Supplementary Fig. 11 ). We did not include other TCGA cancer types in this study because they did not have either the microarray data for co-expression network construction or sufficient prognostic genes identified (due to a limited sample size or inadequate follow-up time). Table 1 Summary of TCGA genomic datasets used in this study. Full size table Co-expression network construction Given Agilent 244 K microarray data for each cancer type, we used the WGCNA package [20] , [21] to build a weighted gene co-expression network that contains 17,813 nodes (genes). The key parameter, β , for weighted network construction was optimized to maintain both the scale-free topology and sufficient node connectivity as recommended in the manual. In such a network, any two genes were connected and the edge weight was determined by the topology overlap measure provided in WGCNA. This measure considered not only the expression correlation between two partner genes but also how many ‘friends’ the two genes shared. The weights ranged from 0 to 1, and reflect the strength of the communication between the two genes. Given a network, we then obtained several key network properties such as the edge weight, node connectivity and modularity. Connectivity was defined as the sum of the weights across all the edges of a node, and the top 1% (or 5%) of the genes with the highest connectivity in the network were defined as hub genes. According to the connectivity distributions, this definition well covered the highly connected nodes in the power-law tails ( Supplementary Fig. 12 ). We obtained the same results when the hub genes were defined based on the adjacency matrix [20] , [21] , in which the edge weight between two gene nodes depended on only their co-expression correlation ( Supplementary Fig. 13 ). We identified the modules using the advanced dynamic tree cut technique, built with the default value of SplitDepth for robust module detection in WGCNA [39] . We obtained the same results when the modules were defined with the SplitDepth value for more sensitive module detection ( Supplementary Fig. 14 ). The co-expression network has been deposited in Synapse (syn1445557). Hub and module analysis of prognostic mRNA genes For each cancer type, we used a Fisher’s exact test to examine the enrichment or depletion of prognostic mRNA or miRNA genes in hub nodes. To examine the cancer-type specificity of the results, we performed the same analysis using hub and prognostic genes from any two cancer types. We used a Fisher’s exact test to evaluate the enrichment of mRNA prognostic genes in modules. To study the conservation of module genes, we defined a score (from 0 to 4) for each gene, with 0 indicating the gene was not a module gene in any of the four cancers, and 4 indicating the gene was a conserved module gene in all four cancer types. We used a Wilcoxon rank sum test with continuity correction to test whether the conservation score was different between prognostic genes and other genes. We considered P <0.05 to be statistically significant. Analysis of prognostic miRNAs and their target genes We first annotated the miRNAs to the corresponding miRNA families and then obtained the predicted conserved targets from TargetScan (Release 6.2) [32] , [40] . For hub analysis, the target genes of all prognostic miRNAs in a cancer type were combined to test the relations with hub genes, as described above. To examine the robustness of the results, target genes with different stringency criteria were used: high-confidence targets were identified as being predicted targets of more than one prognostic miRNA (2–4). For module analysis, we first identified target-module-enriched miRNAs based on whether the target genes of a given miRNA were significantly enriched in at least one module in the co-expression network (FDR<0.1). We then used a Fisher’s exact test to examine whether prognostic miRNAs tended to be target-module-enriched in a given cancer type. Integrative module analysis We used a hypergeometric test to identify prognostic modules as those that are significantly enriched with prognostic mRNAs (FDR<0.1). To assess the clinical relevance of these prognostic mRNA modules, for each cancer type, we classified tumour samples into subtypes (or clusters) based on the expression of module genes (including both prognostic and non-prognostic genes) using non-negative matrix factorization [41] , and then tested the correlations of sample clusters with patient survival using log-rank tests. Similarly, we identified prognostic modules enriched with the target genes of a specific prognostic miRNA (FDR<0.1). We obtained 224 high-confidence significantly mutated genes from TCGA Pan-Cancer Project (syn1750331) and tested their module enrichment in the same way. We used R package ‘topGO’ [42] to annotate modules with GO terms and used IPA (Ingenuity Systems; www.ingenuity.com ) to annotate modules with IPA knowledge-based terms. To identify module correspondence across tumour types, we used a hypergeometric test to examine the pairwise correspondence between any two cross-tumour prognostic modules (FDR<0.1). The results showed great agreement with the cross-tumour module conservation score provided in WGCNA. How to cite this article: Yang, Y. et al. Gene co-expression network analysis reveals common system-level properties of prognostic genes across cancer types. Nat. Commun. 5:3231 doi: 10.1038/ncomms4231 (2014).